Cooperative dynamics in the penetration of a group of intruders in a granular medium An object moving in a fluid experiences a drag force that depends on its velocity, shape and the properties of the medium. From this simplest case to the motion of a flock of birds or a school of fish, the drag forces and the hydrodynamic interactions determine the full dynamics of the system. Similar drag forces appear when a single projectile impacts and moves through a granular medium, and this case is well studied in the literature. On the other hand, the case in which a group of intruders impact a granular material has never been considered. Here, we study the simultaneous penetration of several intruders in a very low-density granular medium. We find that the intruders move through it in a collective way, following a cooperative dynamics, whose complexity resembles flocking phenomena in living systems or the movement of reptiles in sand, wherein changes in drag are exploited to efficiently move or propel. The drag concept in fluid dynamics refers to forces that oppose the relative motion of an object through a fluid [1] , [2] . In the simplest case, when an object moves relatively slow, the drag force is proportional to the velocity. Drag forces become more and more complex as the number of objects increases, and their study has advanced the understanding of the theory of hydrodynamics applied to many-body systems; for example, in the motion of particles or animals in a viscous fluid [3] , [4] , [5] , [6] , [7] , [8] . If the medium is not a fluid but a granular system, drag forces also appear. To understand the resulting dynamics, the impact of projectiles on granular media has been widely studied in the last decades. Normally, an intruder impacting a granular medium penetrates not much deeper than the crater it forms. This shallow penetration highlights the enormous stopping force that a standard medium poses to a colliding object. The crater morphology and the drag dependence, with the impact velocity and depth, density of grains, confinement, packing fraction, among others, have been considered [9] , [10] , [11] , [12] , [13] , [14] , [15] , [16] , [17] . Essentially, the existing granular impact data can be accounted for by the following differential equation: , where m is the mass of the object, g the gravity and η and κ parameters that depend on the material and geometry of the projectile [17] . This knowledge gives us the opportunity to draw important conclusions about geophysical impact events that, by their own nature, are not reproducible. Beyond single-impact experiments, the penetration dynamics of several intruders in a granular medium has never been considered. As far as we know, there is only one work that studies the intruder–intruder and intruder–wall interactions in a granular impact [18] . Although not related with impact cratering phenomena, other authors have investigated the interaction of intruders inside a granular medium under vibration or rotation conditions [19] , [20] , [21] , [22] . In this work, we report how several intruders simultaneously impacting a light granular material [23] , [24] penetrate in a collective way, interacting with each other until they reach a final horizontal configuration. We use a Hele–Shaw cell filled with expanded polystyrene spherical beads (see details in Supplementary Fig. S1 ). During the penetration, different effects are observed, depending on the number of projectiles, initial separation, densities or diameters. However, an intriguing result is that independently of all these factors, the intruders always reach a horizontal line of equilibrium. We propose that this dynamics is due to a continuous change in the local density of the medium that modifies the effective drag forces. Our findings resemble the V-formation of a flock of birds, in which changes in drag are exploited to move in an efficient way. We show that in the realm of low densities, a granular bed at rest has a yield stress so small that it can be easily penetrated as a simple fluid, but it still retains the distinctive properties of its graininess. Dynamics as a function of the number of intruders Before discussing our findings about how a group of intruders penetrate cooperatively the granular medium that is at stake here, it is important to underline two features for the case of a single projectile: first, owing to the low density of the grains, the projectile penetrates up to forty times its own diameter by its own inertia, something never seen in granular penetration experiments (see Supplementary Movie 1 ); second, the dynamics of the projectile is well described by the differential equation cited above, even for these high penetrations (see details in Supplementary Fig. S2 ). These two facts are crucial to understand the cooperative behaviour that emerges when a group of intruders penetrate the medium at the same time. The cooperative dynamics starts to show up when two intruders with the same mass and diameter are launched side by side (see Fig. 1a and Supplementary Movie 2 ). During the impact, they experience a repulsion force that makes them to separate, reaching a maximum separation distance deep inside the cell. Then, they start to attract. 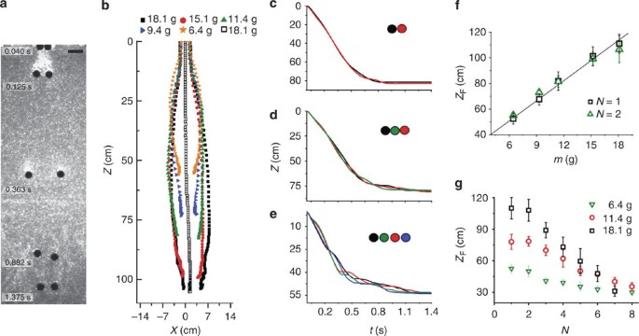Figure 1: Dynamics ofNintruders after a simultaneous impact. (a) Snapshots of the penetration of two intruders in the 2D granular system. The scale bar is 5.0 cm. (b) Trajectoriesx–zfollowed by the intruders for different masses (in grams). (c) A small entanglement at the end of the trajectories is observed in the plotzversust, and this effect is enhanced when the number of intrudersNincreases: (d) Three intruders and (e) Four intruders. The plots correspond tom=11.4 g and the colour of the circles indicates the positions of the intruders in correspondence with their trajectories. (f) Final depthZFversusmfor one and two intruders. (g)ZFas a function ofNfor different masses (D=2.54 cm). In these two plots the error bars correspond to ten repetitions. Figure 1b shows the trajectories x – z of the intruders for different masses (see also Supplementary Fig. S3 ). Note that in all cases, there is repulsion and attraction. Figure 1c shows z versus t for m =11.4 g. Initially, both intruders follow identical vertical trajectories, indicating that they are at the same depth at any given time. At the end, a slight entangling in the trajectories appears, corresponding to the moment in which the intruders start to move slowly and alternately before they stop. The repulsive force appears during the impact. When the disks enter the medium, the grains flow in the outer sides of the pair, reducing the lateral drag force (that is, the lateral pressure). In the centre, on the other hand, the grains are unable to move upwards owing to the intruders' own blockage. Yet, the pressure they produce makes the disks to separate until the material is able to flow freely. About the observed attraction, some clues can be found in the scientific literature to explain its origin [19] , [20] , [21] , [22] . Figure 1: Dynamics of N intruders after a simultaneous impact. ( a ) Snapshots of the penetration of two intruders in the 2D granular system. The scale bar is 5.0 cm. ( b ) Trajectories x – z followed by the intruders for different masses (in grams). ( c ) A small entanglement at the end of the trajectories is observed in the plot z versus t , and this effect is enhanced when the number of intruders N increases: ( d ) Three intruders and ( e ) Four intruders. The plots correspond to m =11.4 g and the colour of the circles indicates the positions of the intruders in correspondence with their trajectories. ( f ) Final depth Z F versus m for one and two intruders. ( g ) Z F as a function of N for different masses ( D =2.54 cm). In these two plots the error bars correspond to ten repetitions. Full size image The entangling in the dynamics is better observed when more than two intruders impact and penetrate the system ( Fig. 1d,e ). It is clear that the greater the number of intruders ( N ), the earlier the entanglement of the trajectories appears and the less the final penetration. Note in Figure 1b that two intruders reach the same depth that an individual intruder with the same mass and V 0 reaches (filled squares and empty squares for intruders of 18.1 g). The same behaviour is obtained for different masses, as shown in Figure 1f , in which the black squares correspond to the penetration of one intruder and the green triangles to the case of two intruders. Figure 1g shows Z F versus N for m =6.4, 11.4 and 18.1 g. The origin of the transition, from N =2 to N ≥3, will be discussed later in the text. To understand the cooperative dynamics that gives rise to the entanglement of the trajectories, let us consider the case of five intruders (see Supplementary Movie 3 ). 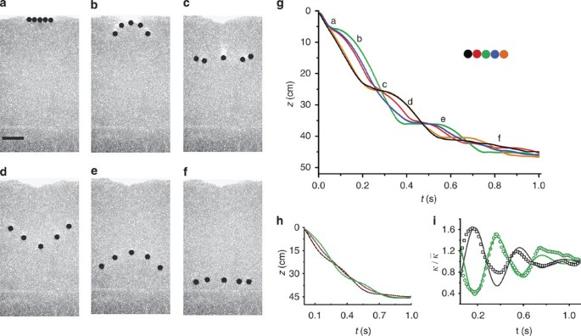Figure 2: Fluttering in granular matter. (a–f) Snapshots of the penetration of five intruders for different time periods: (a) 0.025 s after the impact; (b) at 0.108 s; (c) 0.282 s; (d) 0.361 s; (e) 0.584 s and (f) 0.886 s; see alsoSupplementary Movie 3. The scale bar is 10 cm. (g) The plot showsZversust, where the entanglement of the trajectories is clearly observed. The colour of the circles indicates the positions of the five intruders, in correspondence with their trajectories. (h) The plot shows calculated trajectories using a damped-oscillatory function for the parametersκandη. (i)obtained from the heuristic expression (points) and the fitting function (solid lines) for the intruder in the middle (green) and in the edge (black). The snapshots, as they penetrate the medium, are depicted in Figure 2a–f . The dynamics of the projectiles is clearly cooperative: at t =0 they impact the medium (a). The projectile in the middle stops because the material bellow gets confined by the presence of the lateral intruders, which start to penetrate first (b). They take the lead, fluidizing the material behind them, and, as in the case of two intruders, they repel each other until grains can flow freely. Owing to the flow field produced by the falling partners, the intruder in the centre soon feels a decreased drag. For this reason, it accelerates and now penetrates faster (c). Thereafter, all of them level off deep inside the medium, although this time a bit separated. The process continues with less and less velocity (d and e), and, with a symmetrical fluttering manoeuvre that resembles a flock of birds [5] , [6] , [8] , they finally stop at the same depth (f). Figure 2g shows the z component of the entangled trajectories as a function of time. The curvatures of the plots indicate that the drag force exerted by the medium on each of the disks changes drastically along their trajectories. The entanglement suggests the idea of describing the dynamics of each intruder using the same differential equation employed to analyse the penetration of a single object, but in this case with κ and η that change continuously because of the presence of the whole group. This means that we have to solve a system of five coupled ordinary differential equations (ODEs). However, we can circumvent this difficult task by using a time functional form for the parameters to fit the trajectories. In this case, we use , and a similar expression for η . The experimental trajectories are well fitted, solving the above differential equation with the values k̄ =270 dyn cm −1 , η̄=1.3 g cm −1 and α =2.5 s −2 ( Fig. 2h ). A and ω =2π/τ depend on the intruder under consideration. Figure 2: Fluttering in granular matter. ( a – f ) Snapshots of the penetration of five intruders for different time periods: ( a ) 0.025 s after the impact; ( b ) at 0.108 s; ( c ) 0.282 s; ( d ) 0.361 s; ( e ) 0.584 s and ( f ) 0.886 s; see also Supplementary Movie 3 . The scale bar is 10 cm. ( g ) The plot shows Z versus t , where the entanglement of the trajectories is clearly observed. The colour of the circles indicates the positions of the five intruders, in correspondence with their trajectories. ( h ) The plot shows calculated trajectories using a damped-oscillatory function for the parameters κ and η . ( i ) obtained from the heuristic expression (points) and the fitting function (solid lines) for the intruder in the middle (green) and in the edge (black). 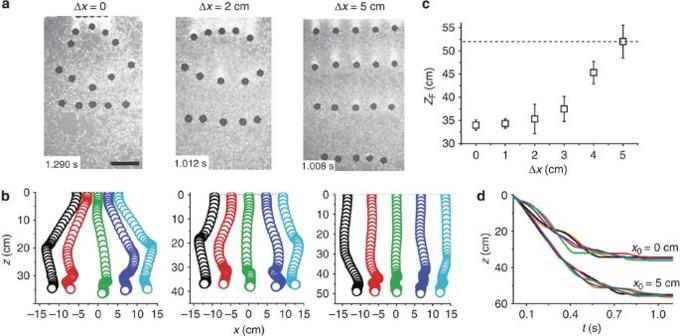Figure 3: Penetration of five intruders for different initial separations Δx. (a) Snapshots of the penetration for Δx=0, 2 and 5 cm,m=6.4 g andD=2.54 cm. (b) Trajectoriesx–zfor the three cases above. (c)ZFversus Δx. The error bars correspond to five repetitions. The dotted line corresponds toZFfor a single intruder with the same mass and diameter. (d)zversustfor two different separations. When Δx=0, the entangling in the trajectories appears right after the impact, but it does not show up when Δx=5 cm. The slight entangling at the end of the trajectories is due to small heterogeneities in the packing fraction. Scale bar, 10 cm. Full size image Z F dependence with the initial separation The cooperative dynamics of the intruders as a function of their initial separation (Δ x ) is shown in Figure 3 for the case of five intruders. In (a) we show snapshots of the intruders ( m =6.4 g and D 1 =2.54 cm) released from rest with different values of Δ x . For Δ x =0, a fluttering behaviour, as the one observed for m =11.4 g in Figure 2a–f , is obtained. When Δ x increases, the fluttering is less and less pronounced (see, for example, the case of Δ x =2 cm). If Δ x >3.0 cm, the intruders practically do not repel and the fluttering disappears (see the complete x – z trajectories in Fig. 3b ). Figure 3c shows that Z F augments with Δ x , up to the value that an individual intruder with the same mass reaches (dotted line). This occurs, as in the case of two intruders, because the interaction only starts to be strong at the end of the trajectories ( Fig. 3d ). If the diameter of the intruders is reduced ( D 2 =0.6 D 1 ), we observe the same behaviour, as Δ x is changed (see Supplementary Fig. S4 ). As in both cases the cooperation disappears when Δ x >3.0 cm, there is no dependence with D . Therefore, we believe that the important size scale to disentangle the trajectories is the diameter of the particles d . Indeed, note that Δ x =3.0 cm ≈ 6 d is approximately the size of an aperture required to have a continuous flow of particles [25] . Then, if the intruders impact the medium with an initial separation Δ x >6 d , the particles can flow freely and there is no initial repulsion. Figure 3: Penetration of five intruders for different initial separations Δ x . ( a ) Snapshots of the penetration for Δ x =0, 2 and 5 cm, m =6.4 g and D =2.54 cm. ( b ) Trajectories x – z for the three cases above. ( c ) Z F versus Δ x . The error bars correspond to five repetitions. The dotted line corresponds to Z F for a single intruder with the same mass and diameter. ( d ) z versus t for two different separations. When Δ x =0, the entangling in the trajectories appears right after the impact, but it does not show up when Δ x =5 cm. The slight entangling at the end of the trajectories is due to small heterogeneities in the packing fraction. Scale bar, 10 cm. Full size image Initial configuration effects The symmetrical entanglement in the penetration is observed only if the group of intruders impacts on the surface horizontally. However, the cooperative dynamics appears independently of the initial configuration. 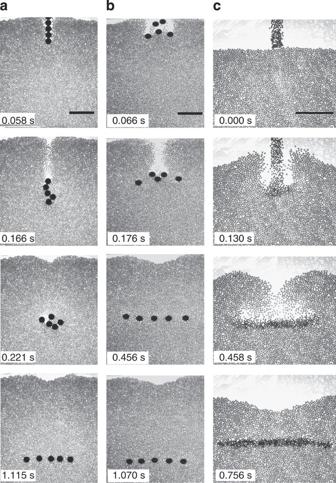Figure 4: Impact and penetration for three different initial configurations. (a) A jet of intruders. First, the jet penetrates the medium vertically. A small fluctuation always causes the disruption of the jet and the intruders start to form a clump. Then, they rearrange themselves slowly and finally stop horizontally. (b) A clump. Independently of the initial positions of the intruders, if they impact the medium together, they descend cooperatively reaching a final horizontal configuration. (c) Small steel particles, impacting as a vertical jet, spread and reach a horizontal configuration. The scale bar is 10 cm in all cases. A jet made with the same five intruders penetrating the bed is shown in Figure 4a . A similar cooperation is observed. Invariably, the intruders loose the vertical formation and start to repel through the mechanism described above, flutter and come to repose always at a horizontal configuration (see Supplementary Movie 4 ). If the intruders are released not like a jet, but as a clump ( Fig. 4b ), the same phenomenon occurs, that is, they repel and cooperatively reach a horizontal array. Even a jet of small steel particles (aspect ratio of 1) penetrating the granular material spreads horizontally, Figure 4c . 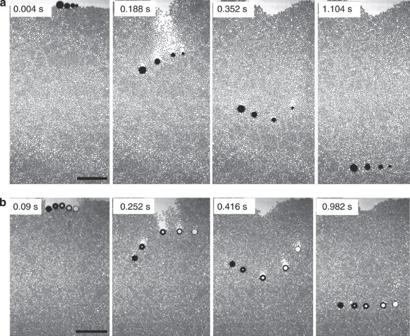Figure 5: Impact and penetration of a heterogeneous group of intruders. (a) Four intruders with the same density (7.8 g ml−1) but different diameters (2.54, 2.04, 1.52 and 1.02 cm, from left to right). (b) Five intruders with the same diameter (2.54 cm) but different densities (7.8, 6.4, 4.9, 4.0 and 2.7g ml−1, from left to right). Scale bar, 10 cm in both cases. Finally, a heterogeneous group of intruders (different densities or diameters), impacting the medium at the same time, would also penetrate cooperatively and deposit themselves on such a horizontal interface (see Figure 5a,b and Supplementary Movie 4 ). The largest (or densest) intruder takes the lead, dragging the group as it descends through the medium. Nonetheless, the full group stops at a final depth between the minimum and maximum distances that single intruders would reach according to their densities and diameters. We show two other examples in Supplementary Figure S5 . Figure 4: Impact and penetration for three different initial configurations. ( a ) A jet of intruders. First, the jet penetrates the medium vertically. A small fluctuation always causes the disruption of the jet and the intruders start to form a clump. Then, they rearrange themselves slowly and finally stop horizontally. ( b ) A clump. Independently of the initial positions of the intruders, if they impact the medium together, they descend cooperatively reaching a final horizontal configuration. ( c ) Small steel particles, impacting as a vertical jet, spread and reach a horizontal configuration. The scale bar is 10 cm in all cases. Full size image Figure 5: Impact and penetration of a heterogeneous group of intruders. ( a ) Four intruders with the same density (7.8 g ml −1 ) but different diameters (2.54, 2.04, 1.52 and 1.02 cm, from left to right). ( b ) Five intruders with the same diameter (2.54 cm) but different densities (7.8, 6.4, 4.9, 4.0 and 2.7g ml −1 , from left to right). Scale bar, 10 cm in both cases. Full size image Because the time dependence of κ and η lies in the constant modification of the local density of the medium as the intruders penetrate and flutter, when their number augments, each one should perceive a greater effective density ( ρ i ) and, therefore, an increased drag. Accordingly, the final penetration depth of the group must decrease when their number increases, as observed in Figure 1g . The change of ρ i is different for each intruder and it depends, as they fall, on the relative positions of the others. Then, a tentative expression for this dependence must consider the fact that the density increases (decreases) if the surrounding intruders are above (below) the projectile in consideration. Moreover, when the shear zones of the intruders do not overlap, ρ i becomes the average local density ρ̄. Such considerations are met with the following heuristic equation (very similar, though, to a hydrodynamic expression used by Crowley [3] , [4] to explain a clumping instability of an array of sedimenting spheres in a viscous fluid): where ( X i , Z i ) and ( X j , Z j ) are the coordinates of the intruder considered and their neighbours, respectively. Θ is the Heaviside function, λ the length of the sheared zone produced by the penetration of the ith intruder (shown in Supplementary Fig. S2 ) and d ij the distance between this and the j th intruder. A i is a free parameter, which is always positive. The sign of the sum term is given by ( Z j – Z i ). Bear in mind that for a group of particles penetrating a fluid, the sum term is negative and the drag always diminishes [3] , [4] Since κ and η are proportional to ρ i [17] , both of them have the same dependence. The above equation is a first approximation to describe the coupling of the ODEs. For the case of five intruders, in Figure 2i , we compare the values of κ obtained using ρ i , as previously indicated (greed circles for the intruders in the middle and squares for intruders in the edge), with those obtained using the damped-oscillatory fitting function (lines). We see that the forms of the curves are quite similar, indicating that our heuristic expression is a good candidate to obtain an explicit coupling of the ODEs that describe the cooperative behaviour observed in the penetration. Note that this model also explains the behaviour observed in Figure 3b . If z i = z j , at all times, each intruder feels the same density, and therefore, reaches the same final penetration depth reached by an individual intruder. Other important aspect is the attraction observed even for Δ x >6 d . This is because of the fact that λ ≫ 6 d , which means that the intruders always feel the flow field of particles. However, the grains are squeezed between the intruders, move faster and therefore a Bernoulli-like effect appears. Now, we can explain the transition observed in Figure 1g when the intruders impact together. For N =2, the final depth is equal to the single case, because there is no lagging between intruders and z i = z j during the most part of the trajectory. For N ≥3, the final penetration is less because the intruders in the middle are left behind or surpass the others, changing the effective density (that is, the drag forces). All in all, we have observed that during penetration a dynamic fluid–solid interface is created by the sinking intruders, and, as their kinetic energy is consumed, this interface evolves to a horizontal line on which the group of intruders finally reach equilibrium (see Supplementary Fig. S6 ). A final configuration other than a horizontal line is improbable because any intruder ahead of the group would always fluidize the medium for the others. Thus, the horizontal array must be the final one. The role of confinement and the density of the medium is now an important issue to address. We claim that the observed phenomena are not privative of two-dimensional (2D) systems. Five identical spheres were launched inside a rectangular container (see Fig. 6a ). The width of the container is three times the diameter of the spheres, but we can still observe the shadow of the balls. Note that in this quasi-3D system, a similar fluttering behaviour is observed (see Supplementary Movie 5 ). The real equivalent phenomenon in the 3D case corresponds to the simultaneous impact of a layer of spheres in a 3D bed: 19 spheres in a hexagonal array ( Fig. 6b ) are released at the same time on the surface of the medium and the moment at which they reach the bottom of the bed ( Fig. 6c ) is filmed. For a column of 30 cm, the 12 intruders of the periphery reach the bottom first ( Fig. 6d ); the second group of 6 intruders arrives later ( Fig. 6e ); and finally, the sphere in the middle arrives ( Fig. 6f ). If the height of the column is changed to 45 cm, the intruders reach the bottom at the same time. Thus, cooperation and fluttering also occurs in a 3D system. 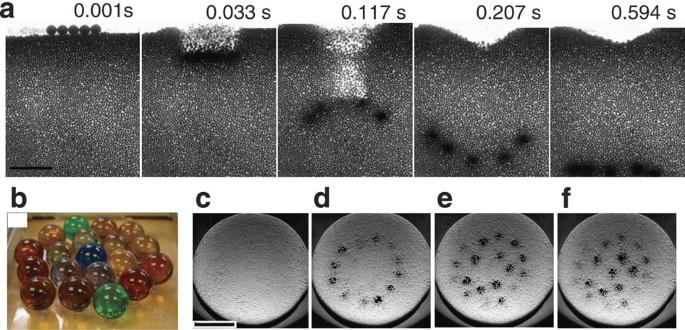Figure 6: Fluttering ofNspheres in a quasi-3D and 3D system. (a) Fluttering of five spheres in a quasi-3D container. The snapshots show the penetration dynamics of five glass spheres in a quasi-3D cell filled with expanded polystyrene beads. This collective behaviour is similar to the one observed for the 2D case. (b) A hexagonal layer of intruders before it is launched in a 3D silo. (c) Bottom view of the silo. (d) The intruders arriving to the bottom; the ones in the periphery are the first to arrive (12 black points att=334.3 ms). (e) Next, the second group arrives (six black points) at 349.8 ms. (f) Finally, the intruder in the middle reaches the bottom at 359.7 ms. Scale bar, (a) 8 cm; (c–f) 15 cm. Figure 6: Fluttering of N spheres in a quasi-3D and 3D system. ( a ) Fluttering of five spheres in a quasi-3D container. The snapshots show the penetration dynamics of five glass spheres in a quasi-3D cell filled with expanded polystyrene beads. This collective behaviour is similar to the one observed for the 2D case. ( b ) A hexagonal layer of intruders before it is launched in a 3D silo. ( c ) Bottom view of the silo. ( d ) The intruders arriving to the bottom; the ones in the periphery are the first to arrive (12 black points at t =334.3 ms). ( e ) Next, the second group arrives (six black points) at 349.8 ms. ( f ) Finally, the intruder in the middle reaches the bottom at 359.7 ms. Scale bar, ( a ) 8 cm; ( c – f ) 15 cm. Full size image Last but not least, the experiments discussed thus far might indicate that the phenomena observed by us need very light beds. However, the penetration of a group of projectiles in standard granular systems would follow the same type of behaviour if the density of the intruders were high enough to fluidize the medium. Indeed, if the polystyrene particles are substituted by glass beads of the same diameter (whose density is 2.3 g ml −1 ), a similar behaviour on the surface is observed (see Fig. 7a ): the large drag present in this type of bed stops the penetrating disks instantaneously, but even so, the array bends. The lateral intruders penetrate more because the glass beads flow at the sides and the intruder in the middle stops for the same reason argued before. However, the intruders do not level off because they cannot further fluidize the medium. If we repeat the experiment in a polystyrene bed using much lighter intruders, the same response is observed (see Fig. 7b ). 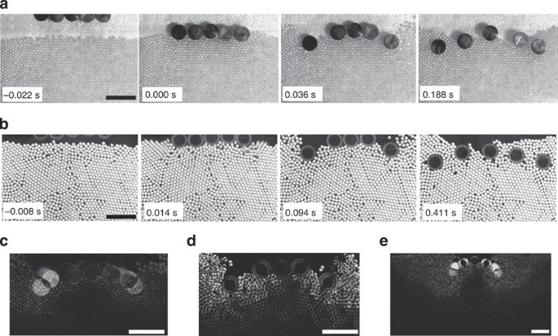Figure 7: Impact with shallow penetration. (a) Impact of five intruders on a glass bed. First, they impact at the same time (t=0 s). Thereafter, the lateral intruders start to penetrate because they fluidize a bit of material, while the intruders in the middle stop because they cannot fluidize (t=0.036 s). They spread on the surface and stop (t=0.188 s). The density ratio of steel/glass is 3.4. (b) A similar behaviour is observed when hollow disks made of Plexiglas impact on a bed of expanded polystyrene beads, wherein the density ratio is 18.4. The fluidization zones on glass (c) and polystyrene beds (d); at the moment of impact. Note that the fluidized zones are very similar. (e) Steel disks penetrating the polystyrene bed, wherein the density ratio is 350. Scale bar, (a–d) 10 cm; (e) 5 cm. Note in Figure 7c,d the similarities in the fluidization surface zones for the above cases, compared with the case in which there is full penetration and fluttering, Figure 7e . Figure 7: Impact with shallow penetration. ( a ) Impact of five intruders on a glass bed. First, they impact at the same time ( t =0 s). Thereafter, the lateral intruders start to penetrate because they fluidize a bit of material, while the intruders in the middle stop because they cannot fluidize ( t =0.036 s). They spread on the surface and stop ( t =0.188 s). The density ratio of steel/glass is 3.4. ( b ) A similar behaviour is observed when hollow disks made of Plexiglas impact on a bed of expanded polystyrene beads, wherein the density ratio is 18.4. The fluidization zones on glass ( c ) and polystyrene beds ( d ); at the moment of impact. Note that the fluidized zones are very similar. ( e ) Steel disks penetrating the polystyrene bed, wherein the density ratio is 350. Scale bar, ( a – d ) 10 cm; ( e ) 5 cm. Full size image In conclusion, we have studied the penetration dynamics of a group of projectiles in a granular medium. The grains are so light that the penetration of the intruders is much larger than in standard granular systems. This large penetration allows us to observe some interesting effects, depending on the number of intruders, composition and initial configurations: (1) two intruders launched side by side repel during the impact and attract during the penetration; (2) if several intruders impact simultaneously, they penetrate the bed following a complex cooperative dynamics in which the interaction among them is mediated by the grains; and 3) Regardless of the way they impact, their sizes or densities, the intruders repel themselves and always distribute along a horizontal line at equilibrium thanks to a fluidization mechanism. This cooperative dynamics, never observed before in granular experiments, might give a clue for advancing the idea that hydrodynamics have an important role in granular systems. Experimental setup The experimental system consists of a vertical 2D cell of 82×120×0.55 cm 3 (width, height and thickness) filled with a monolayer of expanded polystyrene spheres (diameter d =0.5±0.03 cm and density ρ =0.014±0.002 g ml −1 ) purchased at http://www.fanosa.com/ingles/indexingles.html . The container has transparent glass walls to allow filming the frontal face with a high-speed camera (Lightning RDT Plus). These walls have a thickness of 1 cm to avoid deformation and, thus, to obtain the same separation distance through the cell. The walls are cleaned to reduce friction and static charge. The angle of repose of the particles obtained after emptying the material through an opening at the bottom of the cell was 29.67±1.63° for the monolayer, which is a bit higher than the value of 25.68±1.01° for the same material in bulk. As projectiles, we used steel disks with different diameters D and a thickness of 0.52±0.01 cm. Some of them were drilled to produce centred holes of different sizes to obtain different values of mass keeping the diameter constant. At the top of the system, there is a mechanical launching pad to release one or various intruders from rest at the same time. The system is illuminated from behind to obtain a good contrast between the intruder and the medium, and the camera is placed at a distance in which the cell can be completely captured in the visual field. A schematic view of the setup and more details about the properties of the material can be found in Supplementary Figure S1 and Table S1 . Preparation of the system To get similar initial conditions for every launch, the system is prepared before each experiment. First, the cell is put in a horizontal position with a lid on it to avoid loss of material, and air is injected through small holes at the bottom of the cell to distribute the material uniformly. If crystallization is observed, it is reduced with a small steel disk moved through the clusters with a magnet. Then, the system is placed slowly in a vertical position. This procedure guarantees a homogeneous medium with a uniform packing fraction ϕ =0.81±0.01, which is independent of the depth. The values of ϕ were found by measuring the area fraction in a window of 12×12 cm 2 at different depths with the software ImageJ. Finally, the launching pad is centred at the top of the system with the desired intruder configuration. Experiment realization Let us describe a typical experiment involving N intruders. The disks were released together from a height of 5.0±0.5 cm and a video was taken at 1,000 f.p.s. for each launch from the time of the impact until the intruders completely stop. The video was analysed using the software ImageJ to find the positions and velocities of the intruders. The precision time is 1 ms and position resolution is 0.2 cm, defined by 1 pixel size. To eliminate the charge generated by friction between polystyrene particles, they were sprayed with an antistatic product at every ten realizations. For N =2, the experiment was carried out using disks with D =2.54 cm and masses of 6.4, 9.4, 11.4, 15.1 and 18.1 g (2.7, 4.0, 4.9, 6.4 and 7.8 g ml −1 , respectively). The error bars in Figure 1f were obtained from ten repetitions. For N =3, 4 and 5, we used intruders with m =11.4 g. All the Z versus t plots correspond to a single launch. Z F in Figure 1g represents the average penetration depth from the surface to the centre of mass of each intruder, obtained from ten repetitions. In Figure 3 , Δ x corresponds to the distance between the sides of the intruders. Dimensionality and density of the bed In the experiment described in Figure 6a , we used a Plexiglas rectangular container (30×40×6 cm 3 , width, height and thickness, respectively). Five glass spheres ( D =2 cm, m =13.4 g) were released at 5 cm over the surface of the grains. The system was illuminated from behind and a video was taken at 1,000 f.p.s. In Figure 6b , a cylindrical tube (45 cm diameter and 30 cm height) with a transparent Plexiglas plate at the bottom was used. A small steel bolt was glued on top of each of the 19 glass spheres ( D =2 cm, m =13.4 g) and they were distributed in a hexagonal array. The projectiles are held over the surface of the granular medium by an electromagnet, which is turned off to start the free fall of the spheres. A high-speed video (3,000 f.p.s.) of the bottom view was taken to capture the moment at which the intruders arrive. For the snapshots shown in Figure 7a , we used a 2D cell of 40×40×0.55 cm 3 (width, height and thickness) filled with a monolayer of glass spheres (diameter d =0.5 cm and density ρ =2.3 g ml −1 ) and steel disks of m =18.1 g. In Figure 7b the same cell was used, but this time, it was filled with expanded polystyrene spheres. In this case, the intruders were rings of Plexiglas ( d =2.54 cm and ρ =0.257 g ml −1 ). Figure 7c–e were obtained subtracting consecutive frames. How to cite this article: Pacheco-Vázquez, F. & Ruiz-Suárez, J.C. Cooperative dynamics in the penetration of a group of intruders in a granular medium. Nat. Commun. 1:123 doi: 10.1038/ncomms1123 (2010).